Loss of kinesin-14 results in aneuploidy via kinesin-5-dependent microtubule protrusions leading to chromosome cut Aneuploidy—chromosome instability leading to incorrect chromosome number in dividing cells—can arise from defects in centrosome duplication, bipolar spindle formation, kinetochore–microtubule attachment, chromatid cohesion, mitotic checkpoint monitoring or cytokinesis. As most tumours show some degree of aneuploidy, mechanistic understanding of these pathways has been an intense area of research, to provide potential therapeutics. Here we present a mechanism for aneuploidy in fission yeast based on spindle pole microtubule defocusing by loss of kinesin-14 Pkl1, leading to kinesin-5 Cut7-dependent aberrant long spindle microtubule minus-end protrusions that push the properly segregated chromosomes to the site of cell division, resulting in chromosome cut at cytokinesis. Pkl1 localization and function at the spindle pole is mutually dependent on spindle pole-associated protein Msd1. This mechanism of aneuploidy bypasses the known spindle assembly checkpoint that monitors chromosome segregation. Aneuploidy is a hallmark of cancer. Defects in spindle formation and dynamics are known to result in chromosome segregation error resulting in aneuploidy [1] , [2] , [3] , [4] , [5] . The spindle is a machine composed of microtubules (MTs), motors, MT-associated proteins and other regulatory proteins. Kinesin-14 is an important motor organizing the spindle. Kinesin-14, which includes human HSET, Xenopus XCTK2, Drosophila NCD, Saccharomyces cerevisiae Kar3 and Schizosaccharomyces pombe Pkl1, is an MT minus-end-directed motor localized to the spindle poles, which are able to cross-link parallel MTs to focus the spindle pole during mitosis and meiosis, and are able to antagonize kinesin-5, an MT plus end-directed motor localized at the spindle midzone, in a force–balance equilibrium to maintain proper spindle length architecture and function [6] , [7] . Loss of kinesin-14 generally results in chromosome segregation defects [8] , [9] , [10] , [11] , [12] , [13] , or aneuploidy. However, how the loss of kinesin-14 leads to aneuploidy has not been determined. We show in fission yeast that loss of kinesin-14 Pkl1 leads to aberrant spindle pole MT protrusions, resulting from kinesin-5 Cut7 sliding the unfocused pole MTs. Long MT protrusions can subsequently push the post anaphase segregated chromosomes to the site of cell division, resulting in chromosome cut at cytokinesis, thus producing aneuploid cells. pkl1 + deletion results in aberrant spindle MT protrusions Fission yeast S. pombe Pkl1 acts similarly to the metazoan kinesin-14. It is a diffusive MT minus-end-directed motor [14] , localizing at the spindle pole body (SPB) during mitosis [15] , [16] , [17] . Deletion of pkl1 + ( pkl1Δ ) results in unfocused mitotic spindle pole MTs [18] , metaphase spindle length defects [17] , [19] and chromosome segregation defects [16] , [17] . We recently reported that pkl1Δ cells exhibited aberrant spindle MT protrusions [19] . To understand the nature of these protrusions, we performed live-cell imaging of wild-type and pkl1Δ cells expressing mCherry-Atb2 (tubulin) and Sid4-GFP (SPB marker [20] ). We observed spindle MT protrusions in 85% of pkl1Δ cells compared with none in the wild-type cells ( Fig. 1a,c ). The protrusions were parallel to the spindle long axis, appeared during prophase–metaphase, emanated from either one (58% of cells) or both (27% of cells) spindle poles and in most cases were maintained throughout anaphase ( Fig. 1a,c ). Importantly, protrusions came from inside the nucleus. Using Cut11-GFP (nuclear membrane marker [21] ), we observed protrusions pushing out the nuclear envelope and puncturing the envelope when the protrusions were long ( Fig. 1b and see also Supplementary Fig. 3b ), indicating force exertion from the protrusions. 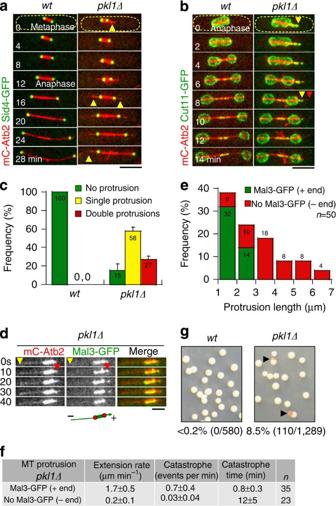Figure 1: Pkl1 maintains SPB integrity. (a) Time-lapse images of wild-type (wt) andpkl1Δcells expressing mCherry-Atb2 (tubulin) and Sid4-GFP (SPB marker) through metaphase and anaphase. Thewtcell has no MT protrusions emanating from the SPB. In contrast, thepkl1Δcell has MT protrusions, which are parallel to the spindle long axis, emanating from one or both SPB (yellow arrow head). The MT protrusion can be long, reaching the cell tip cortex and buckle (time 28 min). Scale bar, 5 μm. (b) Time-lapse images ofwtandpkl1Δcell expressing mCherry-Atb2 and Cut11-GFP (nuclear membrane marker) through anaphase. Thepkl1Δcell has an MT protrusion from inside the nucleus pushing out the nuclear membrane (yellow arrow head, time 0 min). When the MT protrusion reaches a relatively long length, it punctures through the nuclear membrane (red arrow head, time 8 min). Scale bar, 5 μm. (c) Comparative plot of frequency of different MT protrusions inwt(n=20) andpkl1Δ(n=30) cells.wtcells have no aberrant MT protrusions. Bars represent mean±s.d. for multiple experiments. (d) Time-lapse images of a mitotic spindle of apkl1Δcell expressing mCherry-Atb2 and Mal3-GFP (MT plus end-tracking protein EB1). Mal3-GFP is present all along the spindle. Distinct dot of Mal3-GFP tracks the short growing MT (red arrow head, time 10–30 s) and disappears when the MT depolymerizes (time 40 s). The long MT has no Mal3-GFP at its tip (yellow arrow head). Scale bar, 2 μm. (e) Plot of MT protrusion length and polarity frequency inpkl1Δcells. Plus ends are distinguished by Mal3-GFP (green). Minus ends are distinguished by no Mal3-GFP (red). MT protrusions extend from 1 μm (the defined minimum length for reliable measurement) up to 7 μm. Frequencies are pooled from multiple experiments. (f) Comparison of MT dynamic parameters between MT protrusions with and without Mal3-GFP localization at their ends inpkl1Δcells. (See alsoSupplementary Fig. 1). (g) The artificial minichromosome loss assay forwtandpkl1Δcells. Pink colonies represent minichromosome loss. No pink colony is present inwt. About 8.5% ofpkl1Δcolonies are pink. Percentages are pooled from multiple plates. Figure 1: Pkl1 maintains SPB integrity. ( a ) Time-lapse images of wild-type ( wt ) and pkl1Δ cells expressing mCherry-Atb2 (tubulin) and Sid4-GFP (SPB marker) through metaphase and anaphase. The wt cell has no MT protrusions emanating from the SPB. In contrast, the pkl1Δ cell has MT protrusions, which are parallel to the spindle long axis, emanating from one or both SPB (yellow arrow head). The MT protrusion can be long, reaching the cell tip cortex and buckle (time 28 min). Scale bar, 5 μm. ( b ) Time-lapse images of wt and pkl1Δ cell expressing mCherry-Atb2 and Cut11-GFP (nuclear membrane marker) through anaphase. The pkl1Δ cell has an MT protrusion from inside the nucleus pushing out the nuclear membrane (yellow arrow head, time 0 min). When the MT protrusion reaches a relatively long length, it punctures through the nuclear membrane (red arrow head, time 8 min). Scale bar, 5 μm. ( c ) Comparative plot of frequency of different MT protrusions in wt ( n =20) and pkl1Δ ( n =30) cells. wt cells have no aberrant MT protrusions. Bars represent mean±s.d. for multiple experiments. ( d ) Time-lapse images of a mitotic spindle of a pkl1Δ cell expressing mCherry-Atb2 and Mal3-GFP (MT plus end-tracking protein EB1). Mal3-GFP is present all along the spindle. Distinct dot of Mal3-GFP tracks the short growing MT (red arrow head, time 10–30 s) and disappears when the MT depolymerizes (time 40 s). The long MT has no Mal3-GFP at its tip (yellow arrow head). Scale bar, 2 μm. ( e ) Plot of MT protrusion length and polarity frequency in pkl1Δ cells. Plus ends are distinguished by Mal3-GFP (green). Minus ends are distinguished by no Mal3-GFP (red). MT protrusions extend from 1 μm (the defined minimum length for reliable measurement) up to 7 μm. Frequencies are pooled from multiple experiments. ( f ) Comparison of MT dynamic parameters between MT protrusions with and without Mal3-GFP localization at their ends in pkl1Δ cells. (See also Supplementary Fig. 1 ). ( g ) The artificial minichromosome loss assay for wt and pkl1Δ cells. Pink colonies represent minichromosome loss. No pink colony is present in wt . About 8.5% of pkl1Δ colonies are pink. Percentages are pooled from multiple plates. Full size image We next determined the polarity of these protrusions. Using mCherry-Atb2 and Mal3-GFP (MT plus end-tracker EB1 (ref. 22 )), we imaged MT dynamics at 10 s intervals and observed that protrusions showed varied final lengths between 1 and 7 μm long ( Fig. 1d,e ). About 62% of all protrusions were shorter than 3 μm, with three out of four showing Mal3-GFP signal at their ends, indicating plus-end protrusions ( Fig. 1d,e ). The remaining 38% of protrusions were longer than 3 μm and never showed the Mal3-GFP signal at their ends, suggestive of minus-end protrusions ( Fig. 1d,e ). We repeatedly failed to observe bona fide MT minus-end markers such as Alp4-GFP [23] and Mto1-GFP [24] (γ-tubulin complex and associated protein) in these long protrusions. Nevertheless, differential MT dynamics between the short and long protrusions, and Cut7-GFP localization at MT minus ends, indicated that long MT protrusions are probably minus ended. Short MT protrusions showed Mal3-GFP at their ends, extended at rate of V extension =1.7 μm min −1 , persisted growing for T catastrophe =0.8 min, then exhibited frequent catastrophe F catastrophe =0.7 min −1 ( Fig. 1d,f and see also Supplementary Fig. 1a ). In contrast, long MT protrusions showed no Mal3-GFP at their ends, extended at rate of V extension =0.2 μm min −1 , persisted growing for T catastrophe =12 min and exhibited very infrequent catastrophe F catastrophe =0.03 min −1 ( Fig. 1d,f and see also Supplementary Fig. 1b ). Further, recent works showed that the kinesin-5 Cut7 localized to the spindle poles in addition to the spindle midzone [25] and in vitro exhibited minus-end-directed motility [26] . We observed prominent Cut7-3xGFP at the spindle poles of wild-type and pkl1Δ cells ( Supplementary Fig. 1c ). We also observed progressive Cut7-3xGFP accumulation at the ends of the long MT protrusions in pkl1Δ cells ( Supplementary Fig. 1c ). Thus, our result is consistent with long MT protrusions being minus ended. However, we cannot rule out the possibility that long protrusions are somehow more stable plus-ended MTs. We observed that the very long protrusions could reach the cell tip cortex and appeared to push the spindle away from the cell tip ( Fig. 1a and see also Fig. 3c and Supplementary Fig. 3b,c ). The fact that these protrusions form early in mitosis, from inside the nucleus, and parallel to the spindle long axis distinguish them from the cytoplasmic astral MTs, which form only at anaphase and are perpendicular to the spindle long axis [27] . Interestingly, in an artificial minichromosome loss assay [28] , we observed that pkl1Δ cells exhibited 8.5% minichromosome loss, whereas wild-type cells showed <0.2% ( Fig. 1g ). Figure 3: Long MT protrusions lead to chromosome cut at cytokinesis. 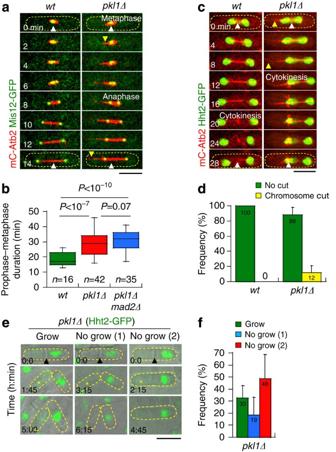Figure 3: Long MT protrusions lead to chromosome cut at cytokinesis. (a) Time-lapse images ofwtandpkl1Δcell expressing mCherry-Atb2 and Mis12-GFP (kinetochore marker) through metaphase and anaphase. The kinetochores separate properly to the opposite spindle poles at anaphase for bothwt(n=50) andpkl1Δ(n=50) cells. Note the appearance of apkl1Δlong MT protrusion (yellow arrow head, time 2 min), which eventually pushes (time 14 min) the associated spindle pole away from the cell tip towards the medial cell division site (white arrow head). Scale bar, 5 μm. (b) Box plot comparing prophase–metaphase duration time ofwt,pkl1Δandpkl1Δ mad2Δmitotic cells. There is no statistical difference (Student’st-test,P=0.07) betweenpkl1Δ(28±8 min) andpkl1Δ mad2Δ(31±6 min) for time to enter anaphase, indicating thatpkl1Δcells do not activate the Mad2-dependent SAC. The shorterwttime to enter anaphase (19±5 min) is possibly due towthaving focused spindle poles, which can form a proper bipolar spindle more quickly33. (c) Time-lapse images ofwtandpkl1Δcells expressing mCherry-Atb2 and Hht2-GFP (histone marker) through anaphase and cytokinesis. Inwt, the spindle separates the segregated chromosome mass to the opposite cell tips, far from the medial cell division site (white arrow head). Inpkl1Δ, the long MT protrusion pushes (yellow arrow head, time 8 min) its associated chromosome mass towards the medial cell division site (white arrow head). Cytokinesis subsequently cuts the misplaced chromosome mass (time 24–28 min), resulting in aneuploidy. Scale bar, 5 μm. (See alsoSupplementary Fig. 3). (d) Comparative plot of frequency of chromosome cut inwt(n=20) andpkl1Δ(n=69) cells. Bars represent mean±s.d. for multiple experiments. (e) Time-lapse bright-field images ofpkl1Δaneuploid cells expressing Hht2-GFP. Three types of aneuploid cell behaviour are observed: ‘grow’, where daughter cells septate and cells receiving more than the typical three chromosomes continues to grow; ‘no grow 1’, daughter cells undergo septation but both do not grow; and ‘no grow 2’, where daughter cells never septate and cells do not grow. Asterisk marks daughter cells with less than three chromosomes. Scale bar, 5 μm. (f) Comparative plot of frequency ofpkl1Δ(n=46) aneuploid cell behaviour. Bars represent mean±s.d. for multiple experiments. ( a ) Time-lapse images of wt and pkl1Δ cell expressing mCherry-Atb2 and Mis12-GFP (kinetochore marker) through metaphase and anaphase. The kinetochores separate properly to the opposite spindle poles at anaphase for both wt ( n =50) and pkl1Δ ( n =50) cells. Note the appearance of a pkl1Δ long MT protrusion (yellow arrow head, time 2 min), which eventually pushes (time 14 min) the associated spindle pole away from the cell tip towards the medial cell division site (white arrow head). Scale bar, 5 μm. ( b ) Box plot comparing prophase–metaphase duration time of wt , pkl1Δ and pkl1Δ mad2Δ mitotic cells. There is no statistical difference (Student’s t -test, P =0.07) between pkl1Δ (28±8 min) and pkl1Δ mad2Δ (31±6 min) for time to enter anaphase, indicating that pkl1Δ cells do not activate the Mad2-dependent SAC. The shorter wt time to enter anaphase (19±5 min) is possibly due to wt having focused spindle poles, which can form a proper bipolar spindle more quickly [33] . ( c ) Time-lapse images of wt and pkl1Δ cells expressing mCherry-Atb2 and Hht2-GFP (histone marker) through anaphase and cytokinesis. In wt , the spindle separates the segregated chromosome mass to the opposite cell tips, far from the medial cell division site (white arrow head). In pkl1Δ , the long MT protrusion pushes (yellow arrow head, time 8 min) its associated chromosome mass towards the medial cell division site (white arrow head). Cytokinesis subsequently cuts the misplaced chromosome mass (time 24–28 min), resulting in aneuploidy. Scale bar, 5 μm. (See also Supplementary Fig. 3 ). ( d ) Comparative plot of frequency of chromosome cut in wt ( n =20) and pkl1Δ ( n =69) cells. Bars represent mean±s.d. for multiple experiments. ( e ) Time-lapse bright-field images of pkl1Δ aneuploid cells expressing Hht2-GFP. Three types of aneuploid cell behaviour are observed: ‘grow’, where daughter cells septate and cells receiving more than the typical three chromosomes continues to grow; ‘no grow 1’, daughter cells undergo septation but both do not grow; and ‘no grow 2’, where daughter cells never septate and cells do not grow. Asterisk marks daughter cells with less than three chromosomes. Scale bar, 5 μm. ( f ) Comparative plot of frequency of pkl1Δ ( n =46) aneuploid cell behaviour. Bars represent mean±s.d. for multiple experiments. Full size image pkl1 and msd1 act together to focus spindle poles The pkl1Δ phenotype of long spindle MT protrusions and minichromosome loss is reminiscent of a similar phenotype reported for deletion of msd1 + ( msd1Δ ) [23] . Msd1 was shown to localize to the spindle poles during mitosis and to interact with the γ-tubulin complex to anchor the MT minus ends at the SPB [23] . The initial report on msd1Δ did not explain how the chromosomes were lost. We examined the relationship between Pkl1 and Msd1. We observed that pkl1Δ , msd1Δ and double-deletion pkl1Δ msd1Δ all exhibited spindle MT protrusions ( Fig. 2a ), and at similar high frequencies ( Fig. 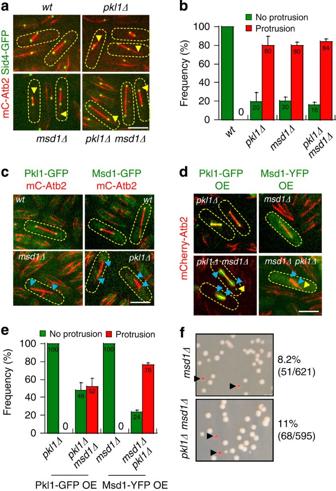2b ), indicating that Pkl1 and Msd1 act in the same pathway. Figure 2: Pkl1 and Msd1 show co-dependent localization to the SPB. (a) Images of mitoticwt,pkl1Δ,msd1Δandpkl1Δ msd1Δcells expressing mCherry-Atb2 and Sid4-GFP. In contrast towt, which have no aberrant MT protrusions,pkl1Δ,msd1Δandpkl1Δ msd1Δ, all have similar short and long MT protrusions (yellow arrow head). Scale bar, 5 μm. (b) Comparative plot of frequency of MT protrusions inwt(n=20),pkl1Δ(n=47),msd1Δ(n=43) andpkl1Δ msd1Δ(n=47) cells.pkl1Δ,msd1Δandpkl1Δ msd1Δcells have similar frequencies of MT protrusions. Bars represent mean±s.d. for multiple experiments. (c) Images of spindle pole localization co-dependency between Pkl1 and Msd1. Inwtcells, both Pkl1-GFP and Msd1-GFP are at the spindle poles. Inmsd1Δcells, Pkl1-GFP is no longer at the spindle pole (blue arrow head). Similarly, inpkl1Δcells, Msd1-GFP is no longer at the spindle pole (blue arrow head). Scale bar, 5μm. (d) Images of Pkl1-GFP overexpression (OE) inpkl1Δandpkl1Δ msd1Δcells, and Msd1-YFP OE inmsd1Δandmsd1Δpkl1Δcells. Pkl1-GFP OE localizes to the spindle and the spindle poles inpkl1Δ, but not the spindle poles inpkl1Δ msd1Δcells (blue arrow head). Msd1-YFP OE localizes to the spindle poles inmsd1Δ, but not inmsd1Δpkl1Δcells (blue arrow head). The absence of Pkl1 or Msd1 results in protrusions (yellow arrow head). Scale bar, 5μm. (e) Comparative plot of frequency of MT protrusion in Pkl1-GFP OE and Msd1-YFP OE cells. Pkl1-GFP OE rescues thepkl1ΔMT protrusion (n=45). Overexpression of Pkl1-GFP inpkl1Δ msd1Δleads to partial rescue of thepkl1Δprotrusion phenotype (n=66), possibly due to Pkl1-dependent MT bundling and focusing ability. Msd1-YFP OE rescues themsd1ΔMT protrusion (n=35). Overexpression of Msd1-YFP inpkl1Δ msd1Δdoes not rescue themsd1ΔMT protrusion phenotype (n=43). Bars represent mean±s.d. for multiple experiments. (See alsoSupplementary Fig. 2). (f) The artificial minichromosome loss assay formsd1Δandmsd1Δ pkl1Δcells. Pink colonies represent minichromosome loss. There is no statistical difference in minichromosome loss amongpkl1Δ(Fig. 1g),msd1Δandmsd1Δ pkl1Δcells (χ2-test,P=0.4). Percentages are pooled from multiple plates. Figure 2: Pkl1 and Msd1 show co-dependent localization to the SPB. ( a ) Images of mitotic wt , pkl1Δ , msd1Δ and pkl1Δ msd1Δ cells expressing mCherry-Atb2 and Sid4-GFP. In contrast to wt , which have no aberrant MT protrusions, pkl1Δ , msd1Δ and pkl1Δ msd1Δ , all have similar short and long MT protrusions (yellow arrow head). Scale bar, 5 μm. ( b ) Comparative plot of frequency of MT protrusions in wt ( n =20), pkl1Δ ( n =47), msd1Δ ( n =43) and pkl1Δ msd1Δ ( n =47) cells. pkl1Δ , msd1Δ and pkl1Δ msd1Δ cells have similar frequencies of MT protrusions. Bars represent mean±s.d. for multiple experiments. ( c ) Images of spindle pole localization co-dependency between Pkl1 and Msd1. In wt cells, both Pkl1-GFP and Msd1-GFP are at the spindle poles. In msd1Δ cells, Pkl1-GFP is no longer at the spindle pole (blue arrow head). Similarly, in pkl1Δ cells, Msd1-GFP is no longer at the spindle pole (blue arrow head). Scale bar, 5μm. ( d ) Images of Pkl1-GFP overexpression (OE) in pkl1Δ and pkl1Δ msd1Δ cells, and Msd1-YFP OE in msd1Δ and msd1Δ pkl1Δ cells. Pkl1-GFP OE localizes to the spindle and the spindle poles in pkl1Δ , but not the spindle poles in pkl1Δ msd1Δ cells (blue arrow head). Msd1-YFP OE localizes to the spindle poles in msd1Δ , but not in msd1Δ pkl1Δ cells (blue arrow head). The absence of Pkl1 or Msd1 results in protrusions (yellow arrow head). Scale bar, 5μm. ( e ) Comparative plot of frequency of MT protrusion in Pkl1-GFP OE and Msd1-YFP OE cells. Pkl1-GFP OE rescues the pkl1Δ MT protrusion ( n =45). Overexpression of Pkl1-GFP in pkl1Δ msd1Δ leads to partial rescue of the pkl1Δ protrusion phenotype ( n =66), possibly due to Pkl1-dependent MT bundling and focusing ability. Msd1-YFP OE rescues the msd1Δ MT protrusion ( n =35). Overexpression of Msd1-YFP in pkl1Δ msd1Δ does not rescue the msd1Δ MT protrusion phenotype ( n =43). Bars represent mean±s.d. for multiple experiments. (See also Supplementary Fig. 2 ). ( f ) The artificial minichromosome loss assay for msd1Δ and msd1Δ pkl1Δ cells. Pink colonies represent minichromosome loss. There is no statistical difference in minichromosome loss among pkl1Δ ( Fig. 1g ), msd1Δ and msd1Δ pkl1Δ cells ( χ 2 -test, P =0.4). Percentages are pooled from multiple plates. Full size image Consistently, in contrast to wild-type cells where Pkl1-GFP and Msd1-GFP localized to the spindle poles [15] , [23] ( Fig. 2c ), Pkl1-GFP was not present at the spindle poles in msd1Δ cells and Msd1-GFP was not present at the spindle poles in pkl1Δ cells ( Fig. 2c ), revealing that both Pkl1 and Msd1 mutually depend on each other to localize at the SPB during mitosis. This suggests that Pkl1, which has very poor processivity in vitro [14] , can localize to the minus end of MT by interacting with Msd1 and the γ-tubulin complex associated with the SPB [15] , [23] , [29] . There, Pkl1 and Msd1 could function together to focus the MT minus ends and with Pkl1 motor heads having additional property of binding adjacent parallel MT minus ends to focus them further. To test this, we overexpressed (OE) Pkl1-GFP in the pkl1Δ and pkl1Δ msd1Δ cells and OE Msd1-YFP in the msd1Δ and msd1Δ pkl1Δ cells ( Fig. 2d ). Pkl1-GFP localized to the spindle and spindle poles in pkl1Δ cells and completely rescued the protrusion phenotype ( Fig. 2c, e ). In pkl1Δ msd1Δ cells, Pkl1-GFP localized to the spindle, but not the spindle poles, and 52% of cells had protrusions ( Fig. 2d,e ). This partial rescue indicates that Pkl1 motor can probably bundle parallel MT minus ends, partially keeping the spindle pole focused. Complementarily, Msd1-YFP OE localized to the spindle poles in msd1Δ cells and completely rescued the protrusion phenotype ( Fig. 2d,e ). However, Msd1-YFP OE did not localize to the spindle poles in msd1Δ pkl1Δ cells and 76% of cells had protrusions ( Fig. 2c,e ), similar to msd1Δ alone ( Fig. 2b ). This indicates that both Pkl1 and Msd1 are required to maintain wild-type spindle poles with wild-type MT focusing. Further, we examined the motor-dead mutant of Pkl1 (Pkl1 md -GFP), where its ATPase activity has been rendered inactive resulting in rigour-binding to MTs [30] . We overexpressed Pkl1 md -GFP in pkl1Δ and pkl1Δ msd1Δ cells. In pkl1Δ cells, Pkl1 md -GFP localized primarily to the spindle poles and almost completely rescued the protrusion phenotype (MT protrusions seen in only 8% of cells; Supplementary Fig. 2a,b ). In contrast, in pkl1Δ msd1Δ cells, Pkl1 md -GFP localized primarily to the spindle and only partially rescued the protrusion phenotype (MT protrusions seen in 51% of cells; Supplementary Fig. 2a,b ). All together, the result confirms that Pkl1 and Msd1 need each other to properly localize to the spindle poles. This tethering at the poles may be critical for focusing MT minus ends at the poles. Further, msd1Δ and double-deletion pkl1Δ msd1Δ both showed similar rates of minichromosome loss compared with pkl1Δ ( Fig. 1f ), with msd1Δ at 8.2% and pkl1Δ msd1Δ at 11% ( Fig. 2f ), consistent with Pkl1 and Msd1 acting in the same pathway. What is the connection between spindle MT protrusions and chromosome loss? Long MT protrusions displace chromosomes for cut at cytokinesis During mitosis, kinetochore-to-MT attachment is established at metaphase and monitored by the spindle assembly checkpoint (SAC); sister chromatid cohesion is severed and the sister chromatids move to the opposite spindle poles during anaphase A; and finally the spindle elongates to separate the segregated chromatids further during anaphase B. Surprisingly, using Mis12-GFP (kinetochore marker [31] ), we observed no kinetochore segregation defects, such as kinetochore lagging indicative of kinetochore-to-MT attachment defects [19] , throughout the different phases of mitosis in pkl1Δ cells ( Fig. 3a ). Deletion of mad2 + , the major component of the SAC [32] , did not shorten the time pkl1Δ cells spent in prophase–metaphase before anaphase ( Fig. 3b ). Interestingly, both pkl1Δ and pkl1Δ mad2Δ cells spent significantly longer time in prophase–metaphase compared with wild-type cells ( Fig. 3b ), probably because pkl1Δ cells, without focused poles, take longer time to organize a bipolar spindle at prophase [33] . All together, these results indicate that the chromosome loss observed in pkl1Δ cells did not arise from defects in the conventional pathways such as SPB duplication, spindle formation, kinetochore-to-MT attachment, chromatid cohesion, or SAC. What then causes chromosome loss in pkl1Δ cells? We reasoned that the long spindle MT protrusions seen in pkl1Δ cells may push the spindle poles and associated segregated chromosomes towards the cell division site, leading to chromosome cut at cytokinesis. Accordingly, in wild-type cells the two chromosome masses labelled with Hht2-GFP (histone marker [34] ) were well separated to the opposite cell tips at the start of cytokinesis ( Fig. 3c )—indicated by the formation of the medial post anaphase array of MTs [27] —and no chromosome segregation defects were observed subsequently. In contrast, in pkl1Δ cells we observed long MT protrusions, which appeared to push—as evident by MT buckling during prolonged contact with the cell tip cortex—its associated chromosome mass to the medial cell division site ( Fig. 3c ). Subsequent cytokinesis appeared to cut through the chromosome mass, resulting in aneuploidy in 12% of mitotic cells ( Fig. 3d ). We further confirmed the chromosome cut phenotype using Cut11-GFP (nuclear membrane marker [21] ). In contrast to wild-type cells, which showed equal segregation of nuclei, pkl1Δ cells with long MT protrusions showed varied combinations of daughter cells with none or two nuclei, and daughter cells with partial nucleus and one nucleus plus micro nucleus ( Supplementary Fig. 3a, b ). We next monitored the long-term fate of the aneuploid cells, specifically where one daughter cell received more than its normal 1N chromosomes. We observed that 67% of aneuploid cells died, either by failure to septate or failure to grow ( Fig. 3e,f ). Interestingly, 33% of aneuploid cells continued growing. Thus, a very small percentage of pkl1Δ cells (4%) will develop into aneuploid cells that can proliferate. Concurrent with long MT protrusions, we observed shorter anaphase spindles in pkl1Δ cells. We compared wild-type and pkl1Δ anaphase B spindle elongation velocity ( Supplementary Fig. 3d,e ). Wild-type anaphase spindles consistently and typically elongated at 0.51±0.04 μm min −1 (mean±s.d., n =13). In contrast, we observed varied spindle velocity in pkl1Δ cells. The majority showed similar velocity as the wild type at 0.50±0.06 μm min −1 ( n =10). These had relatively short MT protrusions between 1 and 2.63 μm, which did not make contact with the cortex, and had no chromosome cut. The second type showed slower velocity at 0.40±0.02 μm min −1 ( n =8). These had MT protrusions between 2.38 and 3.38 μm, which contacted the cortex but had no chromosome cut. Finally, the third type showed very slow velocity at 0.26±0.06 μm min −1 ( n =6). These had protrusions >6 μm, which contacted the cell cortex and exhibited chromosome cut. Thus, there appears to be a negative correlation between spindle length and protrusion length, and there appears to be a positive correlation between protrusion length and chromosome loss ( Supplementary Fig. 3d,e ). The result thus far points to a model of how loss of Pkl1 can lead to aneuploidy ( Fig. 4a ). In wild-type cells, minus ends of parallel MTs are bundled, focused and anchored at the spindle poles by Pkl1 and Msd1. Spindle sliding forces contributed by plus end-directed motors at the spindle midzone can push the spindle poles apart. In the absence of Pkl1 (or Msd1), minus ends of parallel MTs are no longer focused and anchored to the spindle poles [18] , [23] . An unfocused pole would lead to frequent plus-end MT protrusions emanating from the opposite pole. In addition, the pushing forces from the spindle midzone, without a focused pole, would lead to infrequent long MT minus-end protrusions. The very long protrusions would reach the cell tip cortex and push on the post-anaphase segregated chromosome mass at the pole, bringing the chromosomes to the medial cell division site, where on cytokinesis the chromosome mass is cut by the contractile ring. Based on the wild-type fission yeast cell size of 14 μm at mitosis [35] , the MT protrusions would need to be longer than 5 μm, to potentially produce chromosome cut ( Fig. 4a ). This model may explain why very similar percentages of defects were measured in diverse experiments performed on pkl1Δ (or msd1Δ ) cells, for example, 8.5% of cells exhibited minichromosome loss ( Figs 1f and 2f ), 12% of MT protrusions were longer than 5 μm ( Fig. 1e ), to push the chromosome mass to the cut site, and 12% of cells exhibited the chromosome cut phenotype ( Fig. 3d ). 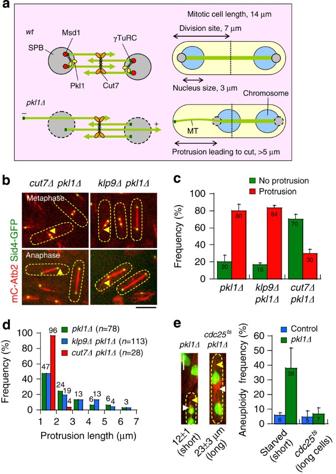Figure 4: Cut7 slides long MT protrusions inpkl1Δcells. (a) Kinesin-14 Pkl1 and Msd1 localize to the SPB, where they can bind to the γ-tubulin complex23,29. Pkl1 can also cross-link parallel minus-end MTs47. Together, they focus the spindle poles during mitosis. In the absence of Pkl1 (or Msd1), the spindle poles are unfocused. Spindle pushing forces from mitotic kinesin-5 Cut7 can then slide minus-end MTs outwards away from the unfocused poles. The long MT protrusions can then push the otherwise properly segregated chromosome to the medial cell division site, resulting in chromosome cut and aneuploidy. Unfocused pole can also lead to short plus-end MT protrusions (coming from the opposite pole). (b) Images ofcut7Δ pkl1Δandklp9Δ pkl1Δcells expressing mCherry-Atb2 and Sid4-GFP in metaphase and anaphase. Only short MT protrusions (yellow arrow head) are present incut7Δ pkl1Δcells. In contrast, both short and long MT protrusions (yellow arrow head) are seen inklp9Δ pkl1Δcells. Scale bar, 5 μm. (See alsoSupplementary Fig. 4). (c) Comparative plot of frequency of MT protrusions inpkl1Δ,klp9Δ pkl1Δandcut7Δ pkl1Δcells. Compared withpkl1Δ(n=50),klp9Δ pkl1Δ(n=65) cells show a similarly high frequency of MT protrusions (χ2-test,P=0.7). In contrast,cut7Δ pkl1Δ(n=50) cells show a significantly lower frequency of MT protrusions (P<10−25). (d) Plot of MT protrusion length distribution frequency inpkl1Δ,klp9Δ pkl1Δandcut7Δ pkl1Δcells. All MT protrusions incut7Δ pkl1Δcells are shorter than 3 μm. In contrast, bothpkl1Δandklp9Δ pkl1Δcells have similar distributions of short and long MT protrusions. Frequencies are pooled from multiple experiments. (e) Comparative plot of frequency of aneuploid cells in short and long mitotic cells.wt(control) andpkl1Δcells were made short by starvation. The average length of short control mitotic cells is 12±1 μm (n=72).cdc25ts(control) andcdc25tspkl1Δcells are made long by overnight growth at 25 °C. The average length of control long mitotic cells is 24±4 μm (n=89). Note thatwtandpkl1Δcells in non-starved growth condition reaches length of 14±1 μm (n=100). Bars represent mean±s.d. for multiple experiments. Figure 4: Cut7 slides long MT protrusions in pkl1Δ cells. ( a ) Kinesin-14 Pkl1 and Msd1 localize to the SPB, where they can bind to the γ-tubulin complex [23] , [29] . Pkl1 can also cross-link parallel minus-end MTs [47] . Together, they focus the spindle poles during mitosis. In the absence of Pkl1 (or Msd1), the spindle poles are unfocused. Spindle pushing forces from mitotic kinesin-5 Cut7 can then slide minus-end MTs outwards away from the unfocused poles. The long MT protrusions can then push the otherwise properly segregated chromosome to the medial cell division site, resulting in chromosome cut and aneuploidy. Unfocused pole can also lead to short plus-end MT protrusions (coming from the opposite pole). ( b ) Images of cut7Δ pkl1Δ and klp9Δ pkl1Δ cells expressing mCherry-Atb2 and Sid4-GFP in metaphase and anaphase. Only short MT protrusions (yellow arrow head) are present in cut7Δ pkl1Δ cells. In contrast, both short and long MT protrusions (yellow arrow head) are seen in klp9Δ pkl1Δ cells. Scale bar, 5 μm. (See also Supplementary Fig. 4 ). ( c ) Comparative plot of frequency of MT protrusions in pkl1Δ , klp9Δ pkl1Δ and cut7Δ pkl1Δ cells. Compared with pkl1Δ ( n =50), klp9Δ pkl1Δ ( n =65) cells show a similarly high frequency of MT protrusions ( χ 2 -test, P =0.7). In contrast, cut7Δ pkl1Δ ( n =50) cells show a significantly lower frequency of MT protrusions ( P <10 −25 ). ( d ) Plot of MT protrusion length distribution frequency in pkl1Δ , klp9Δ pkl1Δ and cut7Δ pkl1Δ cells. All MT protrusions in cut7Δ pkl1Δ cells are shorter than 3 μm. In contrast, both pkl1Δ and klp9Δ pkl1Δ cells have similar distributions of short and long MT protrusions. Frequencies are pooled from multiple experiments. ( e ) Comparative plot of frequency of aneuploid cells in short and long mitotic cells. wt (control) and pkl1Δ cells were made short by starvation. The average length of short control mitotic cells is 12±1 μm ( n =72). cdc25 ts (control) and cdc25 ts pkl1Δ cells are made long by overnight growth at 25 °C. The average length of control long mitotic cells is 24±4 μm ( n =89). Note that wt and pkl1Δ cells in non-starved growth condition reaches length of 14±1 μm ( n =100). Bars represent mean±s.d. for multiple experiments. Full size image cut7 + deletion abolishes long MT protrusions in pkl1Δ cells One prediction from our model is that kinesin-5 Cut7 and/or kinesin-6 Klp9, which localize at the spindle midzone [25] , [36] , provide the sliding forces necessary for minus-end MT protrusion in pkl1Δ cells. Compared with pkl1Δ cells ( Fig. 2a,b ), double-deletion klp9Δ pkl1Δ showed similar short metaphase and long anaphase MT protrusions ( Fig. 4b ), with similar protrusion frequency in 80%–84% of cells ( Fig. 4c ) and similar distribution of protrusion lengths between 1 and 7 μm ( Fig. 4d ). Further, the double-deletion klp9Δ pkl1Δ cells also exhibited long MT protrusion leading to chromosome cut ( Supplementary Fig. 3c ), similar to pkl1Δ cells ( Supplementary Fig. 3b ). In contrast, only 30% of double-deletion cut7Δ pkl1Δ cells exhibited protrusions ( Fig. 4c ) and only short MT protrusions <3 μm throughout metaphase and anaphase ( Fig. 4d ). These short MT protrusions are plus ended, based on Mal3-GFP localization at their ends and their relatively fast MT dynamic parameters ( Supplementary Fig. 4a,b ). We observed only one short MT protrusion in the cut7Δ pkl1Δ cells, which was probably minus ended, based on the absence of Mal3-GFP at its end and its relatively slow MT dynamic parameters ( Supplementary Fig. 4a,b ). Thus, kinesin-5 Cut7, not kinesin-6 Klp9, produces sliding forces from the spindle midzone to push MT minus ends away from the unfocused spindle poles in the absence of Pkl1. In complementary experiments, we showed that the double-deletion cut7Δ msd1Δ cells behaved similarly to cut7Δ pkl1Δ cells. In cut7Δ msd1Δ cells, there were less protrusions compared with msd1Δ ( Supplementary Fig. 4c,d ) and similar frequency of protrusion at 27% of cells compared with cut7Δ pkl1Δ ( Fig. 4c and Supplementary Fig. 4d ), and the protrusions were short, <3 μm long ( Supplementary Fig. 4e ). This further confirms that Pkl1 and Msd1 function in the same pathway at the spindle pole to focus the minus-ended MTs. A second prediction from our model is that cell length probably negatively correlates with protrusion-dependent chromosome loss. An MT can produce pushing forces inversely proportional to the square of its length [37] . Thus, MT protrusions are expected to push more efficiently in short cells compared with that in long cells. We starved wild-type (control) and pkl1Δ cells to create short mitotic cells of 12±1 μm ( n =72) and used cdc25 ts and cdc25 ts pkl1Δ to create long mitotic cells of 23±3 μm ( n =89) ( cdc25 ts is a cell division cycle temperature-sensitive mutation, which blocks cells at the G 2 /M transition, creating long cells [38] ), compared with the typical 14±1 μm ( n =100) length of non-starved log-phase growth of wild-type and pkl1Δ cells. Both the control, short, starved wild-type and the control, long, cdc25 ts cells showed inherent 5%–6% basal level aneuploid cells ( Fig. 4e ). Both short and long cells had spindles and protrusions, which scaled with the cell length ( Fig. 4e ). Nevertheless, the short starved pkl1Δ cells exhibited 38% aneuploidy and the long cdc25 ts pkl1Δ cells exhibited 7% aneuploidy ( Fig. 4e ). Thus, the pkl1Δ MT protrusion-dependent mechanism for aneuploidy is more effective in shorter cell and less effective in longer cells. We identified a potentially new mechanism for aneuploidy in fission yeast. Kinesin-14 Pkl1 and Msd1 localize to the spindle poles and focus the MT minus ends. Their absence leads to pole and MT defocusing, resulting in spindle midzone kinesin-5 Cut7-depedent sliding forces pushing the unfocused MT minus ends away from the spindle poles. Infrequent long MT minus-end protrusions can push the already separated chromosome mass back to the cell centre, where cytokinesis will cut the chromosome mass, creating aneuploid cells. This mechanism is particularly dangerous, because it bypasses the SAC. Further, this mechanism affects small cells more severely than large cells ( Fig. 4a ). In seeming contrast to our findings, an initial electron microscopy (EM) sectioning through one pkl1Δ cell did not observe MT protrusions (but did observe spindle pole and MT minus-end defocusing) [18] . We interpret this to mean that as MT protrusions occurred dynamically in about 80% of pkl1Δ cells, it may require EM sectioning through many cells to catch a protrusion. Consistent with this, EM sectioning through an msd1Δ cell did observe both spindle pole and MT minus-end defocusing, and MT protrusions pushing out the nuclear envelope [23] . Our work is in slight contrast to a recent report on Pkl1 and Cut7 (ref. 39 ). Both works are in agreement with the qualitative findings, for example, pkl1Δ cells have spindle MT protrusions, pkl1Δ cells have chromosome segregation defects and the double-deletion pkl1Δ cut7Δ alleviates the protrusions. However, we are in disagreement concerning the detailed mechanism of function of Pkl1 and Cut7. Olmstead et al . [39] concluded that Pkl1 interacts with the γ-tubulin complex at the spindle poles to inhibit MT nucleation, then Cut7 subsequently interacts with the γ-tubulin complex to remove Pkl1 inhibition of MT nucleation, thus leading to MT protrusions, which occurs outside the nucleus. This interpretation would suggest that all protrusions are probably plus ended. This interpretation cannot explain the key observation that in the presence of Pkl1 (that is, MT nucleation inhibited), spindle MT nucleation still robustly occurred (but no bipolar spindle can form) when Cut7 is deactivated [36] . Our finding favours a different interpretation that the long MT protrusions are probably minus ended. Pkl1 (and Msd1) focuses on the MT minus ends at the poles. Without pole focusing, Cut7 at the spindle midzone can slide some unfocused MTs outwards, resulting in long MT protrusions that are minus ended. Nevertheless, regardless of the polarity of the MT protrusions, only long protrusions can lead to aneuploidy ( Fig. 4a ). In human cells, loss of kinesin-14 HSET [8] , [11] or the MT-associated proteins CLASP1/2 (ref. 40 ) result in spindle pole fragmentation and aneuploidy. It was proposed that spindle sliding forces, in particular by kinesin-5 Eg5, could enhance defects in spindle pole integrity, resulting in chromosome segregation defects [41] . Our current work in fission yeast sheds light on these results and reveals a novel and potentially conserved mechanism for aneuploidy, as all studied proteins are conserved from yeast to human. Aneuploidy can occur due to a lack of kinesin-14 Pkl1-dependent (or Msd1-dependent) spindle pole focusing, causing unfocused force distribution from kinesin-5 Cut7, resulting in long spindle minus-end MT protrusions, which push the chromosome mass to the site of cell division, causing chromosome cut at cytokinesis ( Fig. 4a ). This pathway may be particularly dangerous, as it bypasses checkpoints that ensure chromosome segregation fidelity. A fraction of the resulting aneuploid cells can proliferate [42] and may thus define cancer. Interestingly, cancer cells require kinesin-14 HSET to focus their supernumerary centrosomes into a bipolar-like spindle [43] , as the absence of HSET results in multipolar spindles and subsequent daughter cells die. This suggests that our finding in yeast may not be generalized to human cells. Nevertheless, not enough long-term studies have been done in human cells with inactive HSET to determine whether a small percentage of daughter cells survive and proliferate, as suggested from our current study in fission yeast. Inhibition of kinesin-14 will not be beneficial in the context of cancer therapeutics if some cells survive and proliferate. Strains and media Standard fission yeast media and techniques were used [44] . Gene deletion and fluorescent protein tagging were carried out using a PCR-based protocol [45] . The strains Pkl1-GFP OE and Msd1-YFP OE were under the thiamine-suppressible nmt1-promoter [30] . In the absence of thiamine, cells moderately overexpress Pkl1-GFP and Msd1-YFP after 9–24 h induction. Starved short cells were obtained by growing cells to an optical density of 1.5–2.0. cdc25-22 ts strains were grown at the permissive temperature 25 °C overnight and imaged at an optical density of 0.2–0.6. At the permissive temperature, cdc25-22 ts is inherently longer than wild type. The rigour Pkl1 md -GFP strain was a kind gift from Dr Janet Paluh [30] . Strains used in this study are listed in Supplementary Table 1 . Microscopy Yeast cells were imaged with a Yokogawa spinning-disc confocal microscope equipped with Nikon PlanApo × 100/1.45 numerical aperture or ApoTIRF × 60/1.49 numerical aperture objective lens and a Hamamatsu cooled back-thinned CCD (charge-coupled device) camera or electron multiplying CCD camera [46] . Cells were grown overnight to optical density ∼ 0.5, then placed between 2% agarose YE5S pad and glass coverslip for imaging. Images were acquired at ∼ 20 °C and processed with MetaMorph 7.7 ( www.MolecularDevices.com ). Precise details of imaging conditions are provided for each figure below. Data analysis We defined MT protrusion as MTs parallel to the spindle long axis that extend beyond the SPB for more than 1 μm in length. Experiments were performed at least three times. Data were plotted as bar±s.d. ( n =number) or as Box plots, generated with Kaleidagraph 4.0 ( www.Synergy.com ). Each box encloses 50% of the data with the median value displayed as a line. The top and bottom of each box mark the minimum and maximum values within the data set. Anaphase B spindle lengths were measured by calculating pole-to-pole distances, whose x – y positions were automatically tracked by MTtrackJ plugin in ImageJ ( imagej.nih.gov/ij/ ). Statistical analyses of data were performed in Microsoft Excel 2010 using the Student’s t -test for comparison between means or χ 2 -test for comparison between frequencies. Imaging Figures 1a,b and 2a , Figs 3a,c and 4b,e and Supplementary Figs 1c, 3a,b and 4c : three-dimensional (3D) time-lapse stacks consisting of 11 optical sections of 0.5-μm spacing were collected every 1 min with 500-ms exposure for mCherry and green fluorescent protein (GFP). Figure1d and Supplementary Figs 1a,b and 4a : 3D time-lapse stacks consisting of three optical sections of 0.2-μm spacing were collected every 10 s with 500-ms exposure for mCherry and GFP. Figure 2c : 3D time-lapse stacks consisting of 11 optical sections of 0.5-μm spacing were collected every 1 min with 500-ms exposure for mCherry and 1,500-ms exposure for GFP. Figure 2d and Supplementary Fig. 2a : 3D time-lapse stacks consisting of 11 optical sections of 0.5-μm spacing were collected every 1 min with 700-ms exposure for mCherry and GFP. Figure 3e : 3D time-lapse stacks consisting of 11 optical sections of 0.5-μm spacing were collected every 15 min with 300-ms exposure for mCherry and GFP, plus one snapshot in bright field. Minichromosome loss assay The assay was performed as previously described [28] . The fission yeast strain carrying the artificial S. cerevisiae minichromosome Chr. 16 expressing ADE6 was a kind gift from Dr Takashi Toda. Mutant deletion strains having the ade6-M210 allele were mated with the minichromosome loss strain and progeny cells were selected on adenine minus plates (that is, they contain ADE6 from the minichromosome). Six hundred cells (based on optical density measurements) containing the minichromosome were plated onto selection plates YE4S (adenine minus) and incubated at 30 °C for 3 days. Cells retaining the minichromosome grew white and cells losing the minichromosome grew pink. Total white colonies and pink colonies were counted to provide the percentage of minichromosome loss. How to cite this article: Syrovatkina, V. and Tran, P. T. Loss of kinesin-14 results in aneuploidy via kinesin-5-dependent microtubule protrusions leading to chromosome cut. Nat. Commun. 6:7322 doi: 10.1038/ncomms8322 (2015).